Protein painting reveals solvent-excluded drug targets hidden within native protein–protein interfaces Identifying the contact regions between a protein and its binding partners is essential for creating therapies that block the interaction. Unfortunately, such contact regions are extremely difficult to characterize because they are hidden inside the binding interface. Here we introduce protein painting as a new tool that employs small molecules as molecular paints to tightly coat the surface of protein–protein complexes. The molecular paints, which block trypsin cleavage sites, are excluded from the binding interface. Following mass spectrometry, only peptides hidden in the interface emerge as positive hits, revealing the functional contact regions that are drug targets. We use protein painting to discover contact regions between the three-way interaction of IL1β ligand, the receptor IL1RI and the accessory protein IL1RAcP. We then use this information to create peptides and monoclonal antibodies that block the interaction and abolish IL1β cell signalling. The technology is broadly applicable to discover protein interaction drug targets. Protein–protein interactions are the fundamental functional events that drive all biologic systems at the subcellular and extracellular level. Changes in the specificity and affinity of these interactions can lead to cellular malfunctions and disease [1] . Consequently, the binding interface contact regions between interacting protein partners are important drug targets for the next generation of therapies that block such interactions. Unfortunately, protein–protein interactions have proven to be very difficult pharmacological targets [1] . In fact, many protein–protein interfaces are thought to be undruggable because they are either flat and featureless, or highly complex with multiple three-dimensional (3D) contact points [1] , [2] . In addition, protein–protein binding interfaces often lack catalytic sites [1] , [2] that are the usual basis for drug development. Protein–protein interfaces contain highly conserved amino-acid patches that are hot spots of interaction [3] , [4] , [5] , [6] . Hot spots are preferential drug targets because they contribute the bulk of the coupling stability and the free binding energy of the interaction [4] , [5] . For the vast majority of characterized binary protein–protein interactions, the identity of the two interacting proteins may be known, but the specific amino-acid sequence of their hot-spot region(s) remains unknown [5] . This is because hot spots are difficult and time-consuming to functionally define by existing methods [7] . A major obstacle to hot-spot discovery is that these regions are excluded from solvent contact by a surrounding layer of residues that is analogous to an O-ring [3] . Solvent exclusion favors H bond and salt bridge formation between opposing conserved residues within hot spots [3] , [8] . Other than tomography/crystal structure analysis, current methods cannot directly identify the amino-acid sequence of the physically interacting regions of native proteins, without substantial modification of the interacting proteins by crosslinking (CL) [9] , step-wise mutation or genetic tagging [4] . Thus, there is an important need for an experimental technology that can rapidly reveal the functionally important contact points of native protein complexes in solution. An example of critically important drug target is the three-way interaction of IL1β ligand, its receptor IL1R1 and the accessory protein IL1RAcP. Interleukin signalling requires the interaction of all three proteins [10] , [11] , [12] . In particular, IL1RAcP is an important therapeutic target because it is an indispensable part of the IL1β complex [13] . It stabilizes IL1RI interactions and plays a necessary role in signal transduction. The soluble form of IL1RAcP that contains only the extracellular domain is known to serve as an inhibitor of IL1RI and forms the basis for strategies in which the soluble form of IL1RAcP is administered to inhibit IL1β driven inflammation [13] , [14] . Therapies that block this interaction can be applicable to a variety of diseases, including cancer [15] , rheumatoid arthritis [13] , systemic lupus erythematosus [16] , inflammatory bowel disease [16] , systemic vasculitis [16] , neonatal bronchial dysplasia [13] , neurodegenerative conditions [17] and inflammatory bone and cartilage destruction [18] . Here we introduce a set of small-molecule dyes (molecular paints) that rapidly and tightly coat the exposed surface of protein complexes but do not gain access to the solvent-excluded hot spot(s) between two or more interacting native proteins. Proteolytic enzymes such as trypsin will not cleave the protein regions outside the interface that are painted. Therefore, following proteolysis, peptides for mass spectrometry (MS) will exclusively be generated only from the unmodified opposing regions where the proteins were in intimate contact at the time of the painting. We apply protein painting to sequence and investigate hot-spot regions between the three-way interaction of IL1β ligand, its receptor IL1R1, and the accessory protein IL1RAcP. Our method reveals interface residues associated with opposing tight contact points between the bound ligand and its receptor and the accessory protein. Synthetic peptides and monoclonal antibodies (mAbs) raised against the hidden binding region revealed by protein painting extinguish the three-way interaction of the ligand–receptor–accessory protein complex, and abolish IL1β signal transduction in cultured cells. Protein painting constitutes a new easy to use tool to sequence protein interaction drug targets with high specificity. Rapid paint saturation kinetics and trypsin blockade We identified a panel of small, synthetic aryl hydrocarbon containing organic dyes ( Fig. 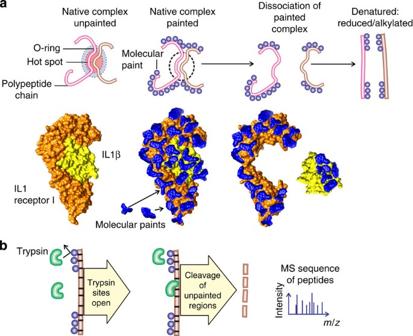Figure 1: Protein painting reveals hidden native hot spots of protein interactions. (a) Paint molecules coat the surface of native protein complexes but cannot gain access to solvent-inaccessible protein–protein interface regions. Interleukin 1β receptor–ligand complex depicted with bound paint molecules to scale. (b) Trypsin cleavage is blocked by the presence of paint molecules that bind non-covalently near trypsin consensus sequences. Following dissociation of painted proteins the area of interaction remains unpainted and is susceptible to trypsin cleavage. Thus, trypsin cleavage peptides will be derived exclusively from unpainted interface areas. 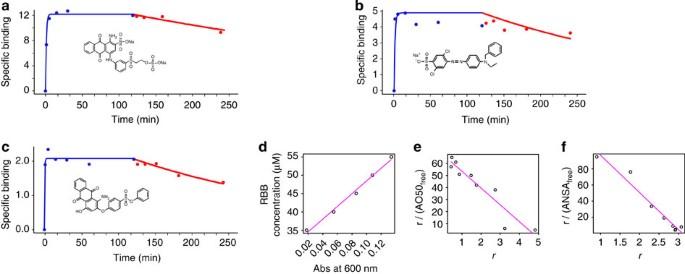Figure 2: Molecular paints rapidly coat native proteins in solution. (a–c) Association (blue) and dissociation (red) binding curves (moles of paint per mole of protein) for paint molecules (structures are shown inset) associating with CA II. Molecular paints have unusually high association rates and low dissociation rates: saturation is reached within 5 min and the off rate is <10% dissociation after 2 h. (d) Calibration data for RBB associated to CA (absorbance spectra for RBB, CA and the complex is reported inSupplementary Fig. 7). (e) Scatchard plot of CA and AO50 shows the number of binding sites to be five, confirming the saturation point of the binding kinetics in (b). (f) Scatchard plot of CA and ANSA shows the number of binding sites to be three. 1 ; Supplementary Figs 1 and 2 ; Supplementary Table 1 ), from a large number of candidate molecules ( Supplementary Table 2 ), that bind to proteins as molecular paints. Paint chemistries were selected because they have extremely rapid on-rates (units: M −1 s −1 ) and very slow off-rates (<10 −5 s −1 , Supplementary Table 1 ) that are 10–100 times higher than most protein–protein interactions [19] , [20] ( Fig. 2 , using at least 10-fold molar excess of dye paint will coat 83% of low-affinity transient interactions that have been characterized [21] , Supplementary Fig. 3 ). Paint chemistries remain bound following protein dissociation or denaturation with 2 M urea ( Fig. 3 ; Supplementary Table 1 ), and bind to multiple sites on the exposed protein surface to achieve complete masking of all the trypsin cleavage sites ( Fig. 4 ; Supplementary Fig. 4 ). Figure 1: Protein painting reveals hidden native hot spots of protein interactions. ( a ) Paint molecules coat the surface of native protein complexes but cannot gain access to solvent-inaccessible protein–protein interface regions. Interleukin 1β receptor–ligand complex depicted with bound paint molecules to scale. ( b ) Trypsin cleavage is blocked by the presence of paint molecules that bind non-covalently near trypsin consensus sequences. Following dissociation of painted proteins the area of interaction remains unpainted and is susceptible to trypsin cleavage. Thus, trypsin cleavage peptides will be derived exclusively from unpainted interface areas. Full size image Figure 2: Molecular paints rapidly coat native proteins in solution. ( a – c ) Association (blue) and dissociation (red) binding curves (moles of paint per mole of protein) for paint molecules (structures are shown inset) associating with CA II. Molecular paints have unusually high association rates and low dissociation rates: saturation is reached within 5 min and the off rate is <10% dissociation after 2 h. ( d ) Calibration data for RBB associated to CA (absorbance spectra for RBB, CA and the complex is reported in Supplementary Fig. 7 ). ( e ) Scatchard plot of CA and AO50 shows the number of binding sites to be five, confirming the saturation point of the binding kinetics in ( b ). ( f ) Scatchard plot of CA and ANSA shows the number of binding sites to be three. 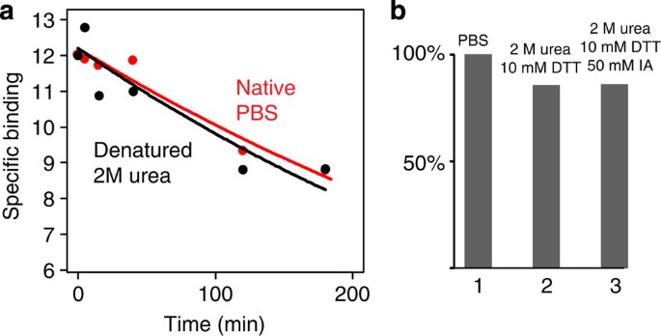Figure 3: Paint molecule coating withstands denaturation. (a) CA was pulsed with RBB and the dissociation kinetics was studied both in native conditions (PBS, red plot) and in denaturing conditions (2 M urea, black plot). The amount of RBB bound to the protein is very similar in the two conditions (bound RBB in 2 M urea >95% of bound RBB in PBS). (b) The amount of RBB bound to CA was compared in native conditions (PBS=100%, column 1), reducing conditions (2 M urea, 10 mM dithiothreitol=86%, column 2) and alkylating conditions (2 M urea, 10 mM DTT, 50 mM iodoacetamide=86%, column 3) after 2 hours of incubation. The conditions tested for this experiment reproduce the experimental steps that are applied to proteins before trypsin digestion for MS and did not show a significant reduction in the amount of dye bound to the denatured reduced and alkylated protein. Full size image Figure 3: Paint molecule coating withstands denaturation. ( a ) CA was pulsed with RBB and the dissociation kinetics was studied both in native conditions (PBS, red plot) and in denaturing conditions (2 M urea, black plot). The amount of RBB bound to the protein is very similar in the two conditions (bound RBB in 2 M urea >95% of bound RBB in PBS). ( b ) The amount of RBB bound to CA was compared in native conditions (PBS=100%, column 1), reducing conditions (2 M urea, 10 mM dithiothreitol=86%, column 2) and alkylating conditions (2 M urea, 10 mM DTT, 50 mM iodoacetamide=86%, column 3) after 2 hours of incubation. The conditions tested for this experiment reproduce the experimental steps that are applied to proteins before trypsin digestion for MS and did not show a significant reduction in the amount of dye bound to the denatured reduced and alkylated protein. 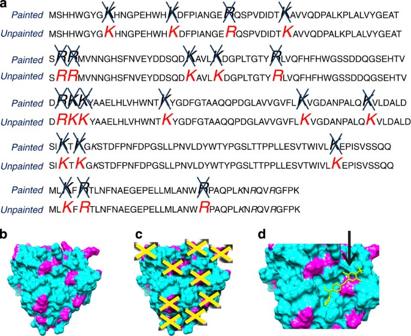Figure 4: Molecular paints block trypsin cleavage sites. (a) Amino acids highlighted in red are consensus trypsin cleavage sites of CA II that were identified by reverse-phase liquid chromatography nanospray tandem MS in the absence of molecular paint (unpainted). Molecular paints (RBB, AO50, R49 and CR) blocked all (100%) consensus trypsin cleavage sites (painted, indicated by a blue X). CA was chosen because it contains 80% of the trypsin cleavage consensus sites that represent all the variations of the amino acids at the carboxy-side of the arginine and lysine. To further confirm that all the possible trypsin cleavage consensus domain were conserved as binding sites for the molecular paints, we conducted similar experiments for aprotinin and albumin in addition to the IL1β-IL1RI-IL1RAcP complex that documented full coverage of all known trypsin cleavage consensus sites for any permissible amino acid. Trypsin cleavage sites are the staple of mass spec sequencing because they mark the protein polypeptide chain at the highest frequency (resolution) compared with other protease cleavage sites40, and they are preferentially distributed on protein surfaces, and in or near previously identified solvent-excluded hot spots3. (b) 3D representation of crystallography structure of CA (PDB no. 1V9E). Surface trypsin cleavage sites are represented in magenta, (c) Yellow crosses indicate trypsin cleavage sites that were blocked by the four molecular paints used (RBB, AO50, R49 and CR). (d) Example representation of AO50 blocking Arg250 on the surface of CA as predicted by docking calculations (SwissDock53, PDB no. 1V9E, ZINC25693528). Full size image Figure 4: Molecular paints block trypsin cleavage sites. ( a ) Amino acids highlighted in red are consensus trypsin cleavage sites of CA II that were identified by reverse-phase liquid chromatography nanospray tandem MS in the absence of molecular paint (unpainted). Molecular paints (RBB, AO50, R49 and CR) blocked all (100%) consensus trypsin cleavage sites (painted, indicated by a blue X). CA was chosen because it contains 80% of the trypsin cleavage consensus sites that represent all the variations of the amino acids at the carboxy-side of the arginine and lysine. To further confirm that all the possible trypsin cleavage consensus domain were conserved as binding sites for the molecular paints, we conducted similar experiments for aprotinin and albumin in addition to the IL1β-IL1RI-IL1RAcP complex that documented full coverage of all known trypsin cleavage consensus sites for any permissible amino acid. Trypsin cleavage sites are the staple of mass spec sequencing because they mark the protein polypeptide chain at the highest frequency (resolution) compared with other protease cleavage sites [40] , and they are preferentially distributed on protein surfaces, and in or near previously identified solvent-excluded hot spots [3] . ( b ) 3D representation of crystallography structure of CA (PDB no. 1V9E). Surface trypsin cleavage sites are represented in magenta, ( c ) Yellow crosses indicate trypsin cleavage sites that were blocked by the four molecular paints used (RBB, AO50, R49 and CR). ( d ) Example representation of AO50 blocking Arg250 on the surface of CA as predicted by docking calculations (SwissDock [53] , PDB no. 1V9E, ZINC25693528). Full size image A pulse of small-molecule paints is applied in vast molar excess to coat native protein preformed complexes ( Fig. 1 ; Supplementary Fig. 5 ). Using a Sephadex G25 molecular sieve quick spin column, saturation binding equilibrium can be reached in 5 min and non-bound paint molecules can be removed in a 1-min column pass-through ( Supplementary Fig. 5 ). When paint molecules are mixed with a native preformed protein complex ( Fig. 1 ; Supplementary Fig. 5 ), the paints non-covalently coat external sites on the protein within minutes, but cannot gain access to the solvent-inaccessible, hidden protein–protein interaction regions ( Fig. 1a ). Each paint molecule spans approximately three amino acids or less ( Supplementary Fig. 1 ). Following protein painting, the unbound paints are removed and the protein–protein interactions are dissociated. This rapid treatment leaves the paint molecules coating all surface trypsin cleavage sites of the protein that were not participating in the interaction interface ( Fig. 1b ). Following painting, the proteins are dissociated, linearized, digested with proteolytic enzymes and sequenced by MS [22] ( Fig. 1b ; Supplementary Fig. 6 ). The paint molecules remain non-covalently bound even after the proteins are reduced and alkylated, and processed for MS sequencing. Following trypsin cleavage of the painted interacting proteins, only the unmodified points of protein partner contact emerge to become available for characterization by MS ( Supplementary Fig. 6 ), ligand-binding assays, or further types of chemical analysis. We can readily differentiate internal solvent-inaccessible residues, within a single protein, from contact points between protein partners, because we separately paint and compare the MS sequence of the native folded proteins before and after they are dissociated. This comparison reveals opposing peptide sequences only found when the proteins are bound together. Screening of paint dyes was performed for individual proteins separately with absorption spectrometry and MS ( Figs 2 and 4 ). Carbonic anhydrase II (CA) was selected as model protein to validate and calibrate the protein-painting method because CA has a large number of widely distributed trypsin cleavage sites comprising >80% of all the possible sequence variations in the specific trypsin recognition sites. The 3D crystal structure of native CA is known, permitting modelling studies of dye-protein binding. CA was pulsed with vast excess of molecule paints disodium; 1-amino-9,10-dioxo-4-[3-(2-sulphonatooxyethylsulphonyl) anilino] anthracene-2–sulphonate (RBB); sodium 4-(4-(benzyl-et-amino)-ph-azo)-2,5-di-cl-benzenesulphonate (AO50); phenyl 4-[(1-amino-4-hydroxy-9,10-dioxo-9,10-dihydro-2-anthracenyl)oxy]benzenesulphonate (R49); 8-Anilino-1-naphthalenesulfonic acid (ANSA) and immediately separated through Sephadex columns. The protein–paint complex was subjected to UV–vis or fluorescence spectrometry in order to determine association–dissociation kinetics and number of binding sites ( Fig. 2 ; Supplementary Fig. 7 ). In order to prove that molecule paints remain bound to proteins during the denaturation process necessary for standard trypsin protocols, CA was pulsed with RBB and the dissociation kinetics was studied both in native conditions (phosphate-buffered saline (PBS); Fig. 3a , red plot) and in denaturing conditions (2 M urea, Fig. 3b , black plot). The amount of RBB bound to the protein is very similar in the two conditions (bound RBB in 2 M urea >95% of bound RBB in PBS). CA was then pulsed with the following paint molecules: RBB, AO50, R49 and disodium; 4-amino-3-[[4-[4-[(1-amino-4-sulphonatonaphthalen-2-yl)diazenyl] phenyl] phenyl] diazenyl] naphthalene-1-sulphonate (CR) and immediately passed through a Sephadex column. MS analysis revealed that this set of four paint molecules remained bound following denaturation and blocked all the trypsin cleavage sites ( Fig. 4 ; Supplementary Fig. 8 ). Hot-spot identification in the interleukin 1 β complex We evaluated the power of protein painting by using it to study the multiple hot spots participating in the three-way interaction of IL1β ligand, its receptor IL1R1 and the accessory protein IL1RAcP ( Fig. 5 ), a critically important drug target. Interleukin signalling requires the interaction of all three proteins [10] , [11] , [12] . Aberrant function of this complex is involved in a variety of diseases, including cancer [15] , rheumatoid arthritis [13] , systemic lupus erythematosus [16] , inflammatory bowel disease [16] , systemic vasculitis [16] , neonatal bronchial dysplasia [13] , neurodegenerative conditions [17] and inflammatory bone and cartilage destruction [18] . 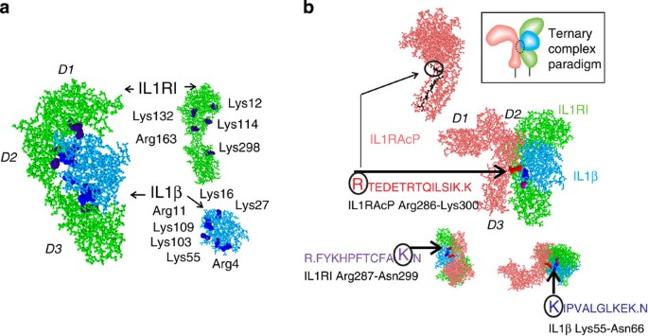Figure 5: Protein painting reveals hot spots between IL1β, IL1RI and IL1RAcP. (a) Identified opposing contact points revealed by the method for the ligand (blue) bound to its receptor (green) before and after dissociation (Fisher exact testP-value<0.0003). Fisher exact test was applied in order to determine whether there was an enrichment of trypsin cleavage sites belonging to protein–protein interface regions among all the trypsin cleavage sites identified by the protein painting method. The total number of trypsin cleavage sites of the two proteins was 49 (26 in the protein–protein interface region). The total number of trypsin cleavage sites identified by the protein painting method was 17, 15 of which belonged to the interface (Fisher exact testP-value<0.0003). (b) IL1RAcP (pink) bound to the receptor (green) ligand (blue) complex. Sequences identified for each protein were found to be opposing and juxtaposed, as noted. The sequence labelled Arg286 (represented in black in the protein model) was used to generate a synthetic peptide antagonist and was used as an antigen for a mouse IgG mAb to Arg286 peptide. Protein painting correctly revealed key contact points with closest proximity obtained by X-ray crystallography and PDBePISA structural analysis software. The two closest interaction points in the three-way complex are IL1RAcP:Arg286–IL1β:Asp54, distance 2.49 Å and IL1RI:Lys298–IL1β:Ser52, distance 2.51 Å (PDB no. 4DEP). These contact points were correctly identified by protein painting in both protein partners. D1, D2 and D3 indicate the domains of IL1RI and IL1RAcP. Figure 5: Protein painting reveals hot spots between IL1β, IL1RI and IL1RAcP. ( a ) Identified opposing contact points revealed by the method for the ligand (blue) bound to its receptor (green) before and after dissociation (Fisher exact test P -value<0.0003). Fisher exact test was applied in order to determine whether there was an enrichment of trypsin cleavage sites belonging to protein–protein interface regions among all the trypsin cleavage sites identified by the protein painting method. The total number of trypsin cleavage sites of the two proteins was 49 (26 in the protein–protein interface region). The total number of trypsin cleavage sites identified by the protein painting method was 17, 15 of which belonged to the interface (Fisher exact test P -value<0.0003). ( b ) IL1RAcP (pink) bound to the receptor (green) ligand (blue) complex. Sequences identified for each protein were found to be opposing and juxtaposed, as noted. The sequence labelled Arg286 (represented in black in the protein model) was used to generate a synthetic peptide antagonist and was used as an antigen for a mouse IgG mAb to Arg286 peptide. Protein painting correctly revealed key contact points with closest proximity obtained by X-ray crystallography and PDBePISA structural analysis software. The two closest interaction points in the three-way complex are IL1RAcP:Arg286–IL1β:Asp54, distance 2.49 Å and IL1RI:Lys298–IL1β:Ser52, distance 2.51 Å (PDB no. 4DEP). These contact points were correctly identified by protein painting in both protein partners. D1, D2 and D3 indicate the domains of IL1RI and IL1RAcP. Full size image We first applied protein painting to the binary interaction between IL1β and its receptor IL1RI (paints used: N-(4-{bis[4-(dimethylamino)phenyl]methylene}-2,5-cyclohexadien-1-ylidene)methanaminium chloride (MV), 3,3′-diethylthiacarbocyanine iodide (DECI), 8-anilino-1-naphthalenesulphonic acid (ANSA) and disodium; 1-amino-9,10-dioxo-4-[3-(2-sulphonatooxyethylsulphonyl)anilino]anthracene-2-sulphonate (RBB)). This revealed interface peptides associated with opposing paint-excluding contact points between the bound ligand and its receptor, and corresponded to the known X-ray crystallography predictions of contact residues [23] ( Fig. 5a ; Supplementary Figs 9–18 ). We next extended protein painting to the receptor, the ligand, and the accessory protein, all painted as a single complex (paints: MV, DECI, ANSA and RBB): our results revealed a three-way candidate hot spot, where all three proteins are in close approximation to each other ( Fig. 5b ), that constitutes a previously unstudied target for potentially blocking IL1β receptor signalling. The MS identified sequences revealed by our method on each separate protein in the complex were all adjacent and juxtaposed to each other based on 3D modelling [12] ( Fig. 5 ). The highly evolutionarily conserved IL1RAcP sequence that emerged (IL1RAcP_Arg286, Supplementary Figs 19–21 ) indicates that the accessory protein, required for interleukin signalling [12] , binds to the receptor–ligand complex in a single very narrow region (orthogonal views, Fig. 5b ). This interaction point incorporating an arginine at the outermost bend of the beta loop is fully consistent with crystallography data [11] , [24] ( Supplementary Fig. 20 ) and can be predicted to participate both in hydrogen bonding and salt bridge formation between the accessory protein and the receptor–ligand complex ( Table 1 ). Consequently, the identification of this beta loop region as a contact point that excludes access to the paints provides new functional information that supports the hypothesis [11] that rotation of the third immunoglobulin domain (D3, Fig. 5b ) in IL1RAcP is necessary for it to touch the composite face of the receptor and ligand (PBD ID# 4DEP). Table 1 Protein painting identified contact points found by crystal structure. Full size table Functionally, hot spots are defined as residues whose mutation to alanine causes the binding free energy (ΔΔ G ) to decrease by at least 2.0 kcal mol −1 (ref. 25 ). For alanine scanning experiments, binding free energy (ΔΔ G ) is calculated as Δ G mut −ΔG wt , where ΔG mut and ΔG wt are the binding free energies upon complex formation of the alanine-mutated and wild-type proteins, respectively [26] . In silico calculations predict that 9.5% of interfacial residues are hot spots [26] . A number of mathematical models have been proposed in order to perform in silico alanine scanning and predict hot-spot energy contributions to total binding energy [27] . The algorithm named Robetta [28] calculates free energy using a physical model that includes a variety of parameters: Lennard Jones interactions, solvation interactions, packing interactions, implicit solvation and hydrogen bonding [28] . Robetta has been demonstrated to achieve a high predictive success (79% of known experimentally found hot-spot residues with a 1.0 kcal mol −1 cutoff, and an average error of 1.06 kcal mol −1 ) [29] . We evaluated the performance of the protein painting method by comparing the specificity of positive peptides found with protein painting to the hot-spot predictions of the Robetta algorithm ( Table 2 ). The Robetta algorithm was applied to the three-protein IL1β-IL1RI-IL1RAcP complex (ΔΔ G complex >1 kcal mol −1 cutoff, pdb#=4DEP, binary interactions: chains A–B, B–C and A–C). A total of 13 out of 15 (87%) proteolytic peptides identified with protein painting contain a hot-spot residue predicted by the Robetta model ( Table 2 ). For this three-protein complex protein painting has a low false-positive rate and a very high specificity (97%=True Negatives/(False Positives+True Negatives=63/(63+2) × 100), see Supplementary Table 3 . Table 2 Protein painting 87% agreement with Robetta-predicted hot spots. Full size table In addition to Robetta (prediction based on energy calculation), we also used two additional prediction tools (KFC2 (ref. 30 ) and Hotpoint [31] ). KFC2 uses machine learning algorithms to find structural patterns that are indicative of hot spots as previously defined [3] ( Supplementary Tables 4 and 5 ) to predict hot spots. Hotpoint is an empirical model based on conservation, accessible surface area, and knowledge-based pair-wise residue potentials of the interface residues [31] . The specificity of protein painting experimentally detected contact solvent-excluded regions was >97% when compared individually with all software methods ( Supplementary Tables 4 and 5 ). 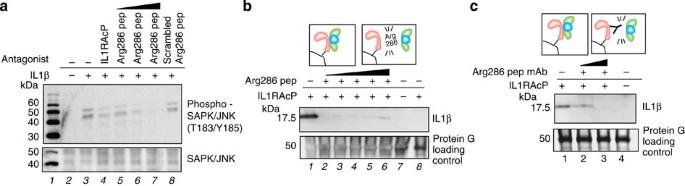Figure 6: IL1RAcP:Arg286 peptide and mAb abolish interleukin signalling. (a) Synthetic antagonist peptide Arg286, identified with protein painting, inhibited SAPK/JNK signalling downstream from IL1RI as effectively as IL1RAcP recombinant protein. In lane 8, scrambled peptide obtained by randomly shuffling Arg286 sequence does not inhibit the signalling downstream from IL1RI. Data are representative of three independent experiments. (b) Arg286 peptide inhibition of ligand pull-down within the receptor complex by His-tagged IL1RAcP. Schematic representation of the complex is depicted in insert. IL1RAcP in the absence of IL1RI does not pull down IL1β, lane 8. (c) Arg286 peptide mAb specific for IL1RAcP peptide extinguishes complex formation depicted in insert. Different software may predict different interaction residues hot spots ( Supplementary Table 6 ). Therefore, protein painting experimental data were compared with the predictions common to all three different computational methods. Protein painting achieved a 93% specificity when compared with the subset of hot-spot predictions common to all the methods ( Supplementary Table 7 ). Functional significance of protein painting findings To test the mechanistic significance of the sequence data ( Tables 1 and 2 ; Fig. 5b ), we treated IL1β-stimulated cells (NCI-ADR-RES [32] ) with synthetic beta loop peptides corresponding to the three-way interface ( Fig. 6a ; Supplementary Figs 19 and 20 ). Synthetic peptides corresponding to the narrow IL1RAcP contact point Arg286 completely blocked IL1β ligand-stimulated signalling in a dose-dependent manner ( Fig. 6a ). To verify that this region was functionally active, we tested whether the peptide blocked the formation of the three-protein complex in vitro ( Fig. 6b ), by pulling down IL1β in the complex through a His-tagged IL1RAcP partner. We found that the Arg286 peptide completely blocked IL1RAcP three-way binding to the receptor–ligand complex ( Fig. 6b ). Finally, to further verify the importance of the IL1RAcP sequence identified by protein painting, we raised a mAb against this region. The mAb blocked the three-protein complex formation in a dose-dependent manner ( Fig. 6b ). Since the Arg286 peptide, or the mAb, acts on opposite faces of the binding site, and can both block pull-down of the ligand–receptor complex, and the peptide itself can substitute for the entire soluble IL1RAcP protein as a competitive inhibitor [13] ( Fig. 6b ), this sequence may be necessary for the interaction of the accessory protein with the other two partners. The Arg286 peptide and/or the mAbs directed against this region constitute novel therapies to potentially block interleukin signalling in vivo . Figure 6: IL1RAcP:Arg286 peptide and mAb abolish interleukin signalling. ( a ) Synthetic antagonist peptide Arg286, identified with protein painting, inhibited SAPK/JNK signalling downstream from IL1RI as effectively as IL1RAcP recombinant protein. In lane 8, scrambled peptide obtained by randomly shuffling Arg286 sequence does not inhibit the signalling downstream from IL1RI. Data are representative of three independent experiments. ( b ) Arg286 peptide inhibition of ligand pull-down within the receptor complex by His-tagged IL1RAcP. Schematic representation of the complex is depicted in insert. IL1RAcP in the absence of IL1RI does not pull down IL1β, lane 8. ( c ) Arg286 peptide mAb specific for IL1RAcP peptide extinguishes complex formation depicted in insert. Full size image We show that protein painting can uncover functionally meaningful sequence regions within hot spots. In the present case of IL1RAcP, protein painting isolated a functionally important binding region and yielded previously unappreciated structural information about the orientation of the IL1RAcP with respect to the other two members of the receptor–ligand complex. While there may be many points of contacts between two interacting proteins, our method highlighted a major single region that is a functionally active target for inhibiting the three protein complex and may provide new strategies for pharmacologic intervention. Comparison with other methods Other methods have been proposed in the past to study interacting proteins. CL chemistry is useful for identifying partners in protein complexes [33] , and the method has been coupled to MS analysis for protein structural modelling [34] . A crosslinker is a molecule with two reactive groups separated by a spacer [34] . A chemical reaction between the crosslinker and the side chain of nearby amino acids (containing primary amines, thiols and carboxylic acids) creates a covalent bond between adjacent residues in a protein complex. The CL reaction can have four different outputs [35] : first, a single peptide bound to a crosslinker molecule with no coupling to another peptide (type 0); second, cyclic or internally bridged peptide (type 1) where the crosslinker reacts with two residues on the same peptide; third, crosslinked peptides (type 2), positive findings in which two peptides are linked and fourth, a combination of the three situations described above (type 3). The crosslinked protein–protein complex is subjected to trypsin and other protease digestion followed by MS analysis. Dedicated software predicts crosslinked peptides based on the following steps: all possible crosslinked peptides are predicted by in silico digestion of protein present in the sample and all possible pair-wise combinations of peptides are calculated [35] . CL may have limitations when the goal is identification of the interaction contact points because the crosslinker molecules, by definition, don’t have access to solvent-excluded interface regions. The output of the CL method is a list of tryptic peptides containing crosslinks. Since both protein painting and CL generate a list of tryptic peptides [34] , we compared the two methods by evaluating the number of positive, and the per cent true positive, tryptic peptides derived from known interface regions ( Table 3 ; Supplementary Table 8 ; Supplementary Figs 22–26 ). Table 3 Comparison of protease-derived fragments with hot-spot predictions. Full size table A second method is hydrogen/deuterium exchange (HDX) [36] . HDX relies on a transient treatment to label amides in the protein backbone with deuterium. Amides in the backbone of proteins in solution are labelled with deuterium by incubation with deuterated (D 2 O) buffers. The hydrogen/deuterium exchange rate depends on the solvent accessibility of amides [37] . Solvent-accessible amides exchange very quickly (within seconds to minutes [36] ), whereas amides that belong to the protein–protein interface are solvent-excluded and will exchange at a lower rate compared with accessible amides The labelling reaction is rapidly quenched at very low pH (2) and low temperature (4 °C) in order to avoid rapid loss of the deuterium label [36] . Proteins are digested at acid pH with pepsin and subjected to MS [36] . Pepsin fragments can be inferred to be derived from interface regions if they show a change in the level of deuterium exchange, reflecting a lower level of solvent accessibility. The MS output of pepsin fragments following HDX is analysed with dedicated software that uses the isotopic distribution and calculates the level of deuterium incorporation [38] . The resolution of the HDX method is a function of the distribution of the pepsin cleavage sites and the proximity of pepsin-derived peptides to solvent-inaccessible regions. The peptide cleavage sites for pepsin are of low specificity and the average size of a pepsin fragment is larger than the 9-amino-acid average size of a trypsin fragment. Nevertheless, it is possible for us to compare the HDX method to protein painting by evaluating the number of positive, and the per cent of true positive, HDX pepsin fragments derived from known interface regions, compared with the same for protein-painting-generated tryptic peptides ( Table 3 ; Supplementary Tables 9 and 10 ; Supplementary Fig. 27 ). A third method is hydroxyl radicals footprinting [39] . Hydroxyl radical footprinting coupled to MS exploits OH radical reaction to map solvent-inaccessible residues in a candidate protein [39] . Unbound and bound proteins are subjected to OH radical reactions and the two outputs are compared with look for peptides that are differentially oxidized [39] Hydroxyl footprinting coupled to MS analysis could be a potential alternative technique for probing protein–ligand interfaces but it requires specialized microfluidics. The OH-radical reaction causes the protein to unfold in milliseconds, exposing residues that are solvent-inaccessible in the native protein [39] . Therefore, a microsecond pulse of laser must be used to cleave hydrogen peroxide and yield hydroxyl radicals that modify proteins before protein unfolding [39] . The specialized experimental apparatus consists of a micro-capillary with a UV transparent window [39] . The reaction mixture containing test proteins, hydrogen peroxide and a scavenger that quenches hydroxyl radicals is irradiated with a laser source coupled to a pulse generator [39] . We have done side-by-side comparison experiments with both CL and HDX ( Supplementary Tables 8–10 ; Supplementary Figs 22–27 ). The data from these experiments, presented in Table 3 , highlight the substantial advantage of protein painting compared with these alternative methods in terms of higher number of total positives, higher per cent of true positives, simplicity and ease of use ( Supplementary Table 11 ). A deuteration time course and specialized temperature control might improve the yield beyond of what is shown in Table 3 . Of note, the critically important binding domain in the three-way IL1β receptor/ligand/accessory protein complex that we identified ( Fig. 5 ) using protein painting was not found by CL or HDX. Our chemistry employs a new principle of solvent exclusion combined with blockade of trypsin recognition sites to functionally identify residues in hot-spot regions that are most tightly associated within the protein complex. According to the O-ring theory of hot spots [3] , [4] , [5] , [6] , [8] , water or solvent is excluded from the hot spot by a surrounding ring of energetically neutral residues. Occlusion of bulk solvent slows dissociation. Our organic dye paint solutions are excluded from entering the hot spot, thereby taking advantage of this principle. Residues that favour both hydrogen bonding and salt bridge formation (Arg, Trp and Tyr) [3] are much more likely to be located within hot spots and these are the same residues that are important for protease (trypsin) recognition and cleavage [40] , compared with other residues (Val, Leu and Ser) [3] . Paints bind with high affinity near trypsin cleavage consensus sites containing charged amino acids such as Arg or Lys, and remain bound after protein partner dissociation, reduction and alkylation ( Figs 3 and 4 ). Using the solvent exclusion principle our method revealed with high concordance the location of hydrogen bonds and salt bridges found with crystallography data ( Table 1 ) at hot-spot contact points ( Table 2 ). Our chemistry works in a manner opposite to chemical CL, which requires solvent-accessible, reactive lysine groups to be available in an appropriate linkable geometry [34] . After screening 23 candidates ( Supplementary Table 2 ), we established a set of 7 small, synthetic aryl hydrocarbon containing organic dyes (see Methods section) that meet the criteria of extremely rapid on rate and low off rate ( Fig. 2 and Supplementary Table 2 ), remain bound following protein dissociation or denaturation ( Fig. 3 ) and block all of the known categories of trypsin cleavage sites ( Fig. 4 ) for any candidate protein that is used for protein painting. The use of the method is very simple and straightforward employing standard MS protocols and software ( Fig. 1 and Supplementary Figs 5 and 6 ). Our method is applied in a short pulse to native preformed protein complexes in solution and the output is the sequence of the solvent-excluded, closely opposed contact points containing trypsin cleavage sites near or at the heart of the hot spot, as shown in Table 2 . The principle of the method introduced here can provide structural and functional information that may not be available with CL, covalent labelling and other tagging methods that have been used to identify members of an interacting protein complex [4] , [9] ( Table 3 ; Supplementary Figs 22–27 ; Supplementary Tables 8–11 ). Prior methods using covalent tagging or CL moieties, by definition, do not enter the solvent-excluded region of protein interaction hot spots. In addition to a high rate of true positives, protein painting offers many advantages compared with other mass-spectrometry-based methods for studying interacting proteins ( Supplementary Table 11 ). While the paint molecules are less than three amino acids, the actual resolution of the hot-spot region we can identify depends on the local density of trypsin cleavage sites (average size of tryptic peptides is nine amino acids [41] ; Supplementary Table 11 ). Based on the results obtained with protein painting, we can calculate the effective distance of the trypsin cleavage site found by protein painting from the closest hot-spot residue predicted by Robetta ( Table 2 ). This distance constitutes the actual resolution of protein painting for the IL1β three-way complex, which is 1.8 amino acids (3, 2, 0, 3, 5, 3, 1, 2, 1, 1, 3, 0 and 0; Table 2 ). Although known hot-spot regions are enriched in charged amino acids comprising trypsin cleavage consensus sites [3] , we may lose resolution for regions with sparse cleavage sites. This limitation is reduced if a sparse region of trypsin residues on one side of the protein–protein interface is compensated by a trypsin cleavage site on the opposite face ( Table 1 ; Supplementary Fig. 20 ). We are currently evaluating the use of additional types of proteinases [41] such as chymotrypsin, or AspN, with overlapping coverage in the hot spot, to further increase the resolution. Structural changes coincident with protein complex formation (ligand binding motion) have been documented to include hinge motion, sheering and shifting [42] . Potentially (but with low likelihood as explained in Supplementary Note 1 ), these structural changes can create solvent-inaccessible sites outside the protein–protein contact domains. Therefore, we cannot exclude that a conformation change occurring after the protein complex has formed will generate a positive hit from protein painting even if the region is not in the interface. All experimental methods aimed at finding solvent-excluded regions in protein complex (hydrogen deuterium exchange [36] , cross-linking [34] and hydroxyl radical footprinting [39] ) encounter the same problem. While this conformation change may not be in the interface it still can be functionally relevant. Thus, it will be valuable for any findings generated by protein painting to be compared with crystallography data, if it exists, for any member of the complex. If crystallography data are not available, an appropriate software [43] might be used to examine whether the solvent-inaccessible sequenced residue is predicted to be outside the binding domain. One important confirmation of the relevance of the region identified with protein painting would be to perform a BLAST analysis in order to check whether the region is evolutionarily conserved. Regions that are functionally important might be expected to be evolutionarily conserved [1] (an example is the identified region RTEDETRTQILSIK discovered using protein painting; Fig. 5 and Supplementary Fig. 21 ). It is theoretically possible that binding of small dye molecules to the outer surface can indirectly change the conformation of the protein partners. Two pieces of evidence support that such an indirect effect on conformation will not substantially affect the ability to find protein–protein contact points and solvent excluding hot spots. First, it has previously been shown for protein-folding time-course studies that a pulse of dye exposure causes a negligible perturbation of the 3D protein conformation after the folding event has taken place [44] . Second, our own studies with the dye paints used herein indicate that a pulse of dye exposure has an undetectable effect on the 3D structure of an already folded protein ( Supplementary Fig. 28 ). We applied protein painting to identify functionally important previously unknown contact points in the three-way interaction of IL1β, IL1RI and IL1RAcP. Recurrent or persistent episodes of inflammation mediated by aberrant activation of IL1β and its receptors characterize a wide spectrum of inflammatory [16] , autoimmune [13] , neoplastic [15] and neonatal disorders [45] . Interaction of IL1β with the extracellular domains of IL1RI and IL1RAcP causes juxtaposition of the intracellular Toll-IL-1 receptor domains of IL1RI and IL1RAcP and triggers intracellular signalling [11] . The IL1R1 extracellular domain binds to IL1β with high affinity, and this is followed by binding of the receptor–ligand complex to IL1RAcP as a necessary step to initiate signalling [11] . IL1β is a monomeric protein constituted by a 12-stranded beta-trefoil domain that does not change substantially after integration into the complex with the receptor and the accessory protein [10] . The extracellular portions of both IL1RI and its family member IL1RAcP are constituted by three immunoglobulin-like domains (D1–D3), generating molecules that resemble a question mark. IL1RI wraps around IL1β like a grasping hand and domains D1, D2 and D3 (forming a concave surface; Fig. 5a ) all contribute to IL1β binding. The IL1β–IL1RI binary complex recruits IL1RAcP and remains virtually unchanged upon binding [10] . IL1RAcP uses the convex surface formed by the D2 and D3 domains to interact with the preformed ligand–receptor complex ( Fig. 5b ) [10] . IL1RI and IL1RAcP are aligned in the complex in an almost perpendicular way. The D1 domain of IL1RAcP points away from IL1β-IL1RI and does not participate in the binding [10] . A rotation of the IL1RAcP D3 domain is necessary for it to touch the IL1β–IL1RI complex [11] . The sequence IL1RAcP_Arg286 belongs to the D3 domain of IL1RAcP and is positioned in the region brought in close proximity to the composite IL1RI–IL1β interface by rotation of the IL1RAcP D3 domain. The requirement for this rotation can explain functional differences between IL1RAcP family members that may be of important disease significance [11] . Thus, IL1RAcP is an important therapeutic target because it is an indispensable part of the IL1β complex ( Fig. 5b ). It stabilizes IL1RI interactions and plays a necessary role in signal transduction. The soluble form of IL1RAcP that contains only the extracellular domain is known to serve as an inhibitor of IL1RI and forms the basis for strategies in which the soluble form of IL1RAcP is administered to inhibit IL1β driven inflammation [13] , [14] . Our results ( Fig. 5 ) uncovered a beta loop at Arg286 of IL1RAcP that excludes the paint molecules and represents a functionally important region. Synthetic peptides mimicking this evolutionarily conserved domain ( Supplementary Fig. 21 ) completely suppressed receptor complex formation and inhibited IL1β signalling ( Fig. 6 ). Moreover, the Arg286 peptide was sufficient to substitute for the entire soluble IL1RAcP molecule as an inhibitor of IL1β signalling. The Arg 286 peptide blocked the three-way complex formation of the receptor partners in solution. To test the functional importance of this region further, we raised a mAb specific for the Arg 286 region, which also inhibited the receptor complex formation ( Fig. 6 ). Previous antibodies studied as IL1β inhibitors [24] bind to a region of the ligand that is not involved in the necessary interaction with IL1RAcP and IL1RI. Thus, the method introduced here has led to the generation of a new class of IL1β-signalling inhibitors that should be studied further in vivo . Our protein painting introduced here can probe protein-binding partners for which little or no interaction region information is known ahead of time, or provide functional information to confirm or extend computational [46] , [47] or analytical approaches (hydrogen deuterium exchange [36] , cross-linking [34] and hydroxyl radical footprinting [39] ). In particular, our chemistry provides a functional approach to discover the subset of opposing residues that are the most closely approximated and thereby may efficiently exclude the solvent and constitute the best drug targets. Future versions of protein painting can also be applied to a population of native proteins containing a subset of interacting members. The direct output will be the amino-acid sequences derived from only the unpainted subset of protein regions that were participating in the protein–protein interactions at the time the paint molecules were introduced, thus comprising a new class of protein interaction information. Molecular painting for MS A series of quantities of CA (Sigma, 10, 20, 30, 50, 65, 80 and 100 pmol in PBS (1 × , Invitrogen)) were preliminarily digested using trypsin and analysed with MS and 65 pmol was chosen as optimal quantity. CA (65 pmol in PBS) was mixed for 5 min with 1000 molar excess of the following molecular paints dissolved in PBS (total volume 50 μl): disodium; 1-amino-9,10-dioxo-4-[3-(2-sulphonatooxyethylsulphonyl) anilino] anthracene-2-sulphonate (RBB; Acros Organics); sodium 4-(4-(benzyl-et-amino)-ph-azo)-2,5-di-cl-benzenesulphonate (AO50) (Sigma); Phenyl 4-[(1-amino-4-hydroxy-9,10-dioxo-9,10-dihydro-2-anthracenyl)oxy]benzenesulphonate (R49) (Sigma); disodium; 4-amino-3-[[4-[4-[(1-amino-4-sulphonatonaphthalen-2-yl)diazenyl] phenyl] phenyl] diazenyl] naphthalene-1-sulphonate (CR) (Sigma). A series of quantities (10, 20, 30, 50, 65, 80 and 100 pmoles in PBS) of interleukin 1β (IL1β, Gibco), interleukin 1 receptor type I (IL1RI, Adipogen), and interleukin 1 receptor accessory protein (IL1RAcP, Novoprotein) were also digested using trypsin and analysed with MS and 65 pmol was chosen as optimal quantity. A total of 65 pmol of unbound IL1β, IL1RI and IL1RAcP were mixed for 5 min with 1000 molar excess of the following 4 molecular paints dissolved in PBS, final volume 50 μl (3 proteins × 4 paints, n =12): N-(4-{bis[4-(dimethylamino)phenyl]methylene}-2,5-cyclohexadien-1-ylidene)methanaminium chloride (MV; Fisher), 3,3′-Diethylthiacarbocyanine iodide (DECI; Sigma), 8-Anilino-1-naphthalenesulphonic acid (ANSA; Sigma) and disodium;1-amino-9, 10-dioxo-4-[3-(2-sulphonatooxyethylsulphonyl)anilino]anthracene-2-sulphonate (RBB; Acros Organics). IL1β (65 pmol in PBS), IL1RI (65 pmol in PBS) and IL1RAcP (65 pmol in PBS) were allowed to interact for 1 hour at room temperature under rotation (total volume 10 μl). Protein complex was mixed for 5 min with 1000 molar excess of the following four molecular paints dissolved in PBS (total volume 50 μl): MV, DECI, ANSA and RBB. All protein–dye solutions were prepared in triplicate and allowed to interact for 5 min, loaded on a size-sieving Sephadex column (mini Quick Spin Oligo Columns, Sephadex G25, Roche) and centrifuged at 1,000 g for 1 min at room temperature. The flow-through was collected, denatured with urea (final concentration 2 M), reduced in 10 mM dithiothreitol (15 min at 37 °C), alkylated with 50 mM iodoacetamide (15 min, room temperature in the dark) and digested with trypsin (Promega) at 1:10 w/w protease/protein ratio for 2 h at 37° C. Solutions were acidified with 6 μl of glacial acetic acid to stop the trypsin reaction. Tryptic peptides were purified by Zip-Tip (Millipore) following manufacturer's instructions, and analysed by reversed-phase liquid chromatography nanospray tandem MS (LC-MS/MS) using an LTQ Orbitrap mass spectrometer (ThermoFisher). MS analysis After sample injection by autosampler, the C18 column (0.2 × 50 mm, Michrom Bioresources, Inc.) was washed for 2 min with mobile phase A (0.1% formic acid) and peptides were eluted using a linear gradient of 0% mobile phase B (0.1% formic acid, 80% acetonitrile) to 50% mobile phase B in 40 min at 500 nl min −1 , then to 100% mobile phase B for an additional 5 min. The LTQ Orbitrap mass spectrometer (Thermo) was operated in a data-dependent mode in which each full MS scan was followed by five MS/MS scans where the five most abundant molecular ions were dynamically selected for collision-induced dissociation using a normalized collision energy of 35%. Tandem mass spectra were searched against the NCBI human and bovine database with SEQUEST using tryptic cleavage constraints. High-confidence peptide identifications were obtained by applying the following filter criteria to the search results: Xcorr versus charge ≥1.9, 2.2, 3.5 for 1+, 2+, 3+ ions; ΔCn>0.1; probability of randomized identification ≤0.01. Analyses of painted dissociated proteins yields a set of peptides (set A) relative to solvent-inaccessible trypsin cleavage sites for each individual protein. Analyses of the preformed protein–protein complex pulsed with paint molecules yields a set of peptide fragments (set B). The difference between set B–set A (solvent-inaccessible trypsin cleavage sites belonging to protein–protein interface regions) is the output of the protein painting method ( Supplementary Fig. 6 ). Association–dissociation kinetics determination To measure the protein–dye equilibrium kinetics [48] , the maximum absorbance for each molecular paint ( Supplementary Fig. 1 ) was identified on a UV-2501PC spectrophotometer (Shimadzu) provided with UV probe 2.10 software in the wavelength region 400-800 nm and using a path length of 1 cm. Spectra for the protein, the molecular paints, and for the bound complex were individually acquired in order to determine whether the binding of molecular paint would shift the maximum absorbance peak of the paint. Calibration was performed as follows (example CA and RBB): considering that CA has multiple binding sites for RBB, it is assumed that within a 35–55 μM concentration (20 μM CAII concentration) all RBB is bound to CAII. Therefore, a linear relationship can be established between the absorbance of the complex and the RBB concentration. Time-course data were modelled with the following equation: Where P is the protein, M is the paint molecule, and PM is the protein–paint molecule complex where [PM] is the concentration of protein-paint molecule complex, t is time, k ass is association constant, [P] is the concentration of protein, [M] is the concentration of paint molecule and k diss is the dissociation constant. The above differential equation yields: Where [PM 0 ] is the concentration of protein–paint molecule complex at time zero, [PM eq ] is the concentration of protein–paint molecule complex at equilibrium, k ass is the association constant, k diss is the dissociation constant, [M] is the concentration of paint molecule and t is time. To study the association kinetics, CA (1 nmole) was mixed with 1000 molar excess of the following molecular paints dissolved in PBS (final volume 50 μl, CA final concentration 20 μM): RBB, AO50, R49 and CR. Protein–paint solutions were allowed to interact for different times (0, 1, 5, 15, 40 and 120 min), loaded on mini Quick Spin Oligo Columns and centrifuged at 1,000 g for 1 min at room temperature. The flow through was collected. The maximum absorbance value of the flow through for the protein–paint complex was registered on the UV-2501PC spectrophotometer at different time points. To study the dissociation kinetics, CA (1 nmol) and molecular paints (RBB, AO50, R49 and CR, 1000 nmol), final volume 50 μl PBS, were allowed to interact for 2 hours and then the unbound paint molecule was separated via mini Quick Spin Oligo Columns. The paint–protein complex was allowed to dissociate for different time periods (1, 5, 15, 40 and 120 min) and then unbound paint molecules were separated via mini Quick Spin Oligo Columns as described above. The bound paint molecule concentration was registered on the UV-2501PC spectrophotometer at different time points. Specific binding is defined as [M bound ]/[P] concentration of bound paint molecule divided by concentration of protein. Specific binding was plotted against time for the association and dissociation kinetics. Non-linear regression calculations to identify the fitted curve of the association and dissociation rates were performed in R software ( http://www.r-project.org/index.html ). Scatchard analysis Scatchard analysis [49] was performed for CA and AO50 in order to confirm the number of binding sites found at saturation in the kinetic experiments. Calibration was performed as described above. Briefly, 10 μM CA was incubated with 0–10 μM AO50. The protein–dye mixture was allowed to interact for 30 min and unbound AO50 was separated via mini Quick Spin Oligo Columns. Absorbance of the complex was measured at 420 nm and correlated to bound AO50 concentration. Scatchard plot was obtained by incubating 10 μM CA with AO50 at increasing concentrations (0, 10, 20, 30, 40, 50, 60, 70, 80, 90 and 100 μM) for 30 min. Unbound AO50 was separated via mini Quick Spin Oligo Columns. Absorbance of the bound dye was measured via absorption spectrometry at 420 nm. ‘ r ’ is defined as the ratio between the concentration of bound dye and the concentration of protein=[AO50bound]/[CA tot ]. A plot of r /[AO50 free ] versus r is built ([AO50 free ] is the concentration of unbound AO50) and a linear relation is fitted. x axis intercept of the fitted line provides an estimate of n (the number of binding sites). For paint molecules that do not have suitable absorbance spectra with maximum peaks separated from protein maximum absorbance peaks, fluorescence spectrometry was used. For the CA/ANSA complex, the same procedure described above and the following excitation and emission wavelength were used λ exc =372 and λ em =471. Emission excitation fluorescence spectra for CA and ANSA were recorded with Jasco Spectrofluorometer FP-8300 and analysed with Jasco Spectra Manager Version 2 software ( Supplementary Fig. 7 ). Crystal structure interface characterization Interface analysis of IL1β–IL1RI and IL1β–IL1RI–IL1RAcP complex structures was performed using the structural analysis module PDBe PISA v1.47 (ref. 50 ; Protein Interface and Assembly) on the PDB entry 1ITB and 4DEP, respectively. Molecular structures were visualized with Swiss-PdbViewer [51] version 4.1. Peptide synthesis and characterization Peptides were custom-produced by Peptide 2.0 Inc. using standard solid phase procedures. Peptide purity (>98%) was assessed by HPLC and MS. Monoclonal antibodies Mouse IgG mAbs (Abmart) were raised against the functionally active portion of IL1RAcPArg286 peptide (TINESISHSRTEDETRTQILS). An immunogenicity-amplified antigen display method was used. Synthetic genes encoding multiple Arg286 peptide epitopes were inserted into a proprietary DNA vector consisting of Immunogenicity Enhancement Factors and DNA sequences. When the vector was expressed in E. coli , particulate, highly immunogenic recombinant proteins that contain multiple Arg286 peptide sequences were produced. Multiple mouse immunizations, multiple fusions and multiple cell line selections were conducted in parallel in order to maximize chances of producing a high-affinity and high-specificity antibody. Resulting antibodies were qualified with (1) solid phase ELISA against Arg286 peptide and selected if they had an ELISA titre higher than 1:100,000, and (2) western blotting and selected if they showed single band reactivity with the IL1RAcP protein (Novoprotein). Cell culture and in vitro inhibition NCI/ADR-RES cells (Division of Cancer Treatment and Diagnosis, National Cancer Institute) were cultured in Dulbecco’s modified Eagle’s medium (Gibco) with 10% fetal bovine serum (ATCC), and 2 mM L-glutamine (ATCC) at 37 °C, 5% CO 2 , in a humidified environment. NCI/ADR-RES cells (2 × 10 6 cells per well) were plated into six-well tissue culture dishes. The following day, cells were pre-treated for 30 min with soluble IL1RAcP (1 μg ml −1 ) lacking the trans-membrane domain, Arg286 peptide (TINESISHSRTEDETRTQILS, 8, 41 and 81 μg ml −1 ) and a scrambled peptide obtained by randomly shuffling Arg286 sequence (HLRNISRISSITDTSETETEQ, 81 μg ml −1 ). Cells were washed with Dulbecco’s modified Eagle’s medium with 10% fetal bovine serum, and 2 mM glutamine and were stimulated with IL1β at 10 ng ml −1 for 30 min. Following incubation, cells were washed in ice-cold PBS, incubated with 100 μl of cell lysis buffer (10% Bond Breaker TCEP solution (Thermo Scientific), 45% T-PER tissue protein extraction reagent (Thermo Scientific) and 45% Novex Tris–Glycine SDS sample buffer 2 × (Invitrogen)), scraped, transferred to Eppendorf tubes, and heated at 100 °C for 10 min. Cell lysates were analysed by western blotting. Immunoprecipitation of IL1β three-way complex IL1β (0.44 μg ml −1 ), IL1RI (2 μg ml −1 ) and 6xHis-tagged IL1RAcP (Abcam, 0.72 μg ml −1 ) were incubated with Arg286 peptide (16, 8, 4, 2 and 1 μg ml −1 ) in 50 μl of PBS for 1 hour at room temperature under rotation. In parallel, IL1β, IL1RI and 6xHis-tagged IL1RAcP were allowed to interact without Arg286 peptide as a positive control. IL1β and 6xHis-tagged IL1RAcP were allowed to interact in the absence of IL1RI as a negative control. After 1 h, protein mixtures were incubated with magnetic beads decorated with anti-6His mouse mAb obtained as follows. BcMag Protein G Magnetic Beads (50 μl, Bioclone) were washed three times with washing buffer (57.7 mM Na 2 HPO 4 , 42.3 mM NaH 2 PO 4 , pH 7.0) and incubated with anti-6xHis mouse mAb (0.4 mg ml −1 , Abcam) for 30 min under rotation. Magnetic beads were separated from the supernatant with neodymium magnets, washed three times with washing buffer (57.7 mM Na 2 HPO 4 , 42.3 mM NaH 2 PO 4 , pH 7.0) and incubated with protein mixtures for 1 hour at room temperature under rotation. Magnetic beads were separated from the supernatant with neodymium magnets and washed three times with washing buffer (57.7 mM Na 2 HPO 4 , 42.3 mM NaH 2 PO 4 , pH 7.0). Immuno-precipitated proteins were eluted with 20 μl of 4 × sample buffer (10 min, 70 °C). Immuno-precipitated proteins were analysed by western blotting. Western blotting Proteins were separated by 1D gel electrophoresis in 4–20% Tris–Glycine gel in the presence of Tris–Glycine SDS running buffer (125 V, 90 min) and then transferred onto Immobilion PVDF membrane. The membrane was blocked with PBS supplemented with 0.2% (w/v) I-Block and 0.1% Tween 20 for 1 h at room temperature, and then incubated with anti-phospho-SAPK/JNK (T183/Y185), SAPK/JNK or IL1β antibodies (1:1,000, Cell Signaling Technology) overnight at 4 °C under continuous agitation. After washes with PBS supplemented with 0.2% I-Block (w/v) and 0.1% Tween 20, the detection method was species-specific horseradish-peroxidase-conjugated anti-IgG secondary antibody (Invitrogen) chemiluminescence system (ECL Plus, Pierce). The protein blot was imaged using a Kodak 4000MM. BLAST analysis To confirm that the IL1RAcP peptide (TINESISHSRTEDETRTQILS) selected by our protein painting method was conserved among species, a BLAST search was performed with Protein Basic Local Alignment Search Tool (pblast) available at http://blast.ncbi.nlm.nih.gov/Blast.cgi?CMD=Web&PAGE_TYPE=BlastHome . CL reactions IL1β, IL1RI and IL1RAcP were dissolved in 20 mM HEPES buffer (pH7.7) at a 2 μM concentration. A total of 130 pmol of each protein was mixed and allowed to form a complex for 1 h at room temperature. DST (Thermo Scientific) and sulpho-EGS (Thermo Scientific) solutions in dimethyl sulphoxide (DMSO, Fisher) were freshly prepared at a concentration of 10 mM. DST and sulpho-EGS were added to protein mixtures in a 100 molar excess and volume of the solution was brought to 200 μl. CL reactions were allowed to proceed for two time periods (30 and 120 min, total experimental conditions=2 crosslinkers × 2 time periods=4). A control without CL was prepared in the same fashion. Aliquots of 100 μl were taken after 30 and 120 min and the CL reaction was terminated by adding 5 μl of a 400 mM NH 4 HCO 3 solution. Samples were denatured with urea (final concentration 2 M), reduced in 10 mM dithiothreitol (15 min at 37 °C), alkylated with 50 mM iodoacetamide (15 min, room temperature in the dark) and digested with trypsin (Promega) at 1: 10 w/w protease/protein ratio for 2 h at 37 °C. Solutions were acidified with 6 μl of glacial acetic acid. Tryptic peptides were purified by Zip-Tip (Millipore) following the manufacturer’s instructions and analysed by reversed-phase LC-MS/MS using an LTQ Orbitrap mass spectrometer (ThermoFisher). MS analysis was performed as described above. Data obtained from MS were analysed with StavroX (ref. 52 ). Hydrogen/deuterium exchange Deuterium off-exchange measurements were performed on the IL1β three-way complex in order to identify interface regions of the interacting proteins and compare the results with the protein painting method. Preliminarily, pepsin digestion was performed on IL1β, IL1RI and IL1RAcP in order to identify peptic peptides. Briefly, 400 pmol of each protein in 120 μl of water containing 5 μl of 2% TFA (final pH=2) was digested by adding 50 μl of pepsin immobilized on 6% agarose beads (2.5 mg ml −1 , Pierce) for a duration of 10 min on ice with mixing every minute in order to avoid agarose gel beads precipitation. The pepsin–agarose beads were washed twice before use with 1 ml of chilled 0.1% TFA by vortexing and centrifugation (2 min, 7 r.c.f., 4 °C). The immobilized pepsin was removed by centrifugation (1 min, 14 r.c.f., 4 °C) and peptic fragments were analysed by MS. Proteins were individually subjected to deuterium on-exchange reaction and were used as positive controls. Peptic fragments of deuterated proteins were obtained in triplicate as described below. Stock solution of deuterated Tris buffer was prepared as follows: 1 M Tris buffer (pH 7.9) was lyophilized and re-suspended in D 2 O (Cambridge Isotope laboratories). Lyophilized proteins (IL1β, IL1RI and IL1RAcP) were diluted in 25 mM Tris D 2 O, pD 7.9 at a concentration of 100 μM. A total of 400 pmol (in 12 μl total volume) of the three proteins were individually deuterated for 10 min at room temperature. Each sample was quenched by addition of 120 μl of H 2 O containing 5 μl of 2% TFA (final pH=2) on ice. Samples were digested by adding 50 μl of washed pepsin–agarose slurry for a duration of 10 min on ice with mixing every minute. The immobilized pepsin was removed by centrifugation (1 min, 14 r.c.f., 4 °C). The supernatant was divided into aliquotes and immediately frozen at −80 °C. In a separate set of experiments, proteins were individually deuterated, allowed to interact and then deuterium was off-exchanged as described below. Regions that retained the deuterium label are indicative of solvent-excluded surface areas participating in protein–protein interactions. On-exchange experiment was performed on each protein separately, in triplicate as described above. Briefly, 400 pm (in 4 μl) of the three proteins were individually deuterated for 10 min at room temperature. The three proteins were combined and allowed to complex for 2 min (total volume 12 μl). The off-exchange reaction was initiated by the addition of 115 μl of H 2 O and allowed to proceed for 10 min at room temperature. Samples were quenched with 5 μl of 2% TFA (final pH=2) on ice. Samples were immediately digested as described above by adding 50 μl of pepsin slurry for a duration of 10 min on ice with mixing every minute. Pepsin beads were removed by centrifugation (1 min, 14 r.c.f., 4 °C). The supernatant was divided into aliquotes and immediately frozen at −80 °C. MS analysis was performed within 24 h from the freezing time for all the samples. Data analysis of MS output was performed with Mass Spec studio, an upgraded version of the Hydra software [38] that was kindly provided by Dr Schriemer. Docking Docking of CA-AO50 was performed with SwissDock web service [53] (PDB no. 1V9E, ZINC25693528). Docking results were visualized with Chimera 1.8 (ref. 54 ). How to cite this article: Luchini, A. et al . Protein painting reveals solvent-excluded drug targets hidden within native protein–protein interfaces. Nat. Commun. 5:4413 doi: 10.1038/ncomms5413 (2014).